Stabilizing lithium–sulphur cathodes using polysulphide reservoirs The possibility of achieving high-energy, long-life storage batteries has tremendous scientific and technological significance. An example is the Li–S cell, which can offer a 3–5-fold increase in energy density compared with conventional Li-ion cells, at lower cost. Despite significant advances, there are challenges to its wide-scale implementation, which include dissolution of intermediate polysulphide reaction species into the electrolyte. Here we report a new concept to mitigate the problem, which relies on the design principles of drug delivery. Our strategy employs absorption of the intermediate polysulphides by a porous silica embedded within the carbon–sulphur composite that not only absorbs the polysulphides by means of weak binding, but also permits reversible desorption and release. It functions as an internal polysulphide reservoir during the reversible electrochemical process to give rise to long-term stabilization and improved coulombic efficiency. The reservoir mechanism is general and applicable to Li/S cathodes of any nature. Lithium–sulphur (Li–S) batteries [1] are one of the most promising candidates to couple renewable energy sources for green transportation and large-scale energy storage owing to their various desirable characteristics including competitive cost, and low environmental impact. Moreover, their high theoretical energy density is over 5 times larger than that of conventional Li-ion batteries based on intercalation electrodes [2] . Despite these advantages, massive implementation of Li–S batteries remains hindered by various challenges that mainly arise from the cathode. The major problem is rapid capacity fading, which is mainly due to dissolution of polysulphide anions (S n 2− )—intermediate reaction species formed on charge and discharge—from the cathode into the electrolyte [3] , [4] . Once the polysulphide ions diffuse out from the nanostructured cathode, not only will their reaction with the Li anode cause active mass loss, but also the redeposition of sulphide species from the electrolyte back onto the cathode surface generates large agglomerates at the end of discharge. The polysulphide anions also act as an internal redox shuttle, which gives rise to low coulombic efficiency: namely, a charge capacity larger than the corresponding discharge capacity [5] . Various electrolyte systems have been employed to solve the problem, including polymers [6] . A physical barrier that prevents diffusion of the polysulphide species could solve the dissolution problem, but in the long term this could be compromised. A fast-responding sulphur battery requires facile transport of electrolyte/Li + into and out of the sulphur electrode, but eventually some soluble polysulphide ions will diffuse over the physical barrier, which initiates the shuttle phenomenon. Recently, there has been some promising progress made on new sulphur battery configurations. Li 2 S has been employed as an initial active material [7] in the sulphur electrode, to couple with non-metallic lithium anodes, that is, graphite [8] , a carbon/tin alloy [9] and Si nanowires [10] . These sulphur batteries still suffer capacity loss, however, due to the untackled polysulphide dissolution problem. Cobalt polysulphides have been investigated as cathode materials to reduce the solubility of polysulphide ions in the electrolyte [11] . Efforts devoted to electrolytes include rational selection of solvents [12] and introduction of additives such as LiNO 3 (ref. 13 ), which diminishes the effect of the polysulphide shuttle mechanism as a result of complex reactions on the Li metal anode. Ordered mesoporous carbons have been employed as nanosized reaction chamber assemblies for the sulphur electrode [14] . This approach overcomes the low conductivity of the sulphur electrode, but falls short of completely controlling polysulphide dissolution. Our group has developed a polymer-decorated mesoporous carbon/sulphur-interwoven nanocomposite as a sulphur cathode, where the surface polymer chains can effectively retard the polysulphide anion dissolution [15] . Importantly, the agglomeration of precipitated sulphides on the cathode is greatly reduced. This is important because such a build-up on the surface results in capacity fading owing to poor contact with the conductive carbon surface underneath, and the barrier to Li-ion diffusion that is created. With all these considerations in mind, it is still vital to retain the polysulphide anions within the cathode layer by using additional methods. On-site adsorption is one promising concept. Oxide additives, including Mg 0.6 Ni 0.4 O (ref. 16 ) and Al 2 O 3 (ref. 17 ) nanoparticles (~50 nm), were employed as adsorbents in the sulphur cathode and they showed some effect to increase an otherwise low coulombic efficiency; however, the effect of these additives can only be observed at a low level of sulphur loading in the cathode, which is probably due to their limited adsorption surface area. Additives based on porous carbons have also been described [18] . However, electronically conductive additives will facilitate the reduction of the polysulphides to insoluble sulphides onto their surface during the charge cycle. Once the adsorbents are covered, their function ceases. A successful additive should not only be inert to redox reactivity and show strong absorption capacity, but also allow facile desorption of the polysulphide anions. Herein, as a significant step towards solving the challenge of polysulphide dissolution, we present a new approach to sulphur cathode composites that comprise a carbon–sulphur nanocomposite together with a small fraction of a mesoporous silica additive. We were inspired by studies using triblock copolymer-templated SBA-15 as a reversible drug delivery system. SBA-15 is a well-developed mesoporous silica that exhibits high surface area, large pore volume, bi-connected porous structure and highly hydrophilic surface properties [19] . These characteristics allow it to adsorb certain kinds of drugs and release them in a highly reproducible and predictable manner. It has been shown that both small and large molecular drugs can be entrapped within the mesopores by an impregnation process and liberated via a diffusion-controlled mechanism [20] . Although the Si–O groups that cover its internal surface are too weak to engage in molecular drug interaction without being first functionalized, they serve as ideal binding sites for the sulphur cathode. The cavities not only accommodate polysulphide anions through weak binding via the positively charged silica surface, but also permit reversible desorption. Thus, they function as an internal sulphide reservoir to absorb and release the active material for electrochemical reduction–oxidation during cycling. We employed SBA-15 with a platelet morphology, that not only exhibits good absorption properties but can also be easily dispersed with carbon–sulphur particles. Other silicas with suitable pore sizes, such as zeolite beta or MCM-41—which have also been employed for targeted drug delivery [21] —should be equally effective. Furthermore, we have developed and utilized a new large-pore (>10 nm) porous carbon for the sulphur/carbon nanocomposite to illustrate the efficacy of the SBA-15 additive in binding the polysulphide anions. Polysulphide diffusion is more of a concern in highly open pore systems than in CMK-3/S [15] , which was examined previously, and hence it necessitates an effective absorption additive. An additional benefit is that this combination can offer better rate performance owing to faster kinetics as we show herein. Synthesis and characterization of the mesoporous carbon (SCM) The mesoporous carbon was prepared by replicating a silica monolith. This methodology was originally reported by Jaroniec et al . [22] , [23] and is modified in this study. The monolith is formed by drying a commercialized silica colloid (LUDOX HS-40 40wt%, Sigma-Aldrich). 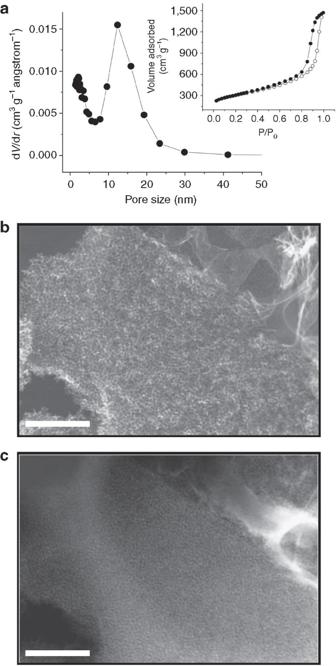Figure 1: Porosity characterization of the 'silica colloidal monolith'-derived mesoporous carbon (SCM). (a) Pore size distribution for SCM carbon. Inset: adsorption/desorption isotherm; (b) high-resolution SEM image of SCM; (c) dark-field STEM image of SCM. (b,c) Scale bar=300 nm. The mesoporous carbon prepared from it by the replica technique is referred to as SCM (silica colloidal monolith), which exhibits the N 2 absorption and desorption isotherm shown in Figure 1a . SCM exhibits a Brunauer-Emmett-Teller (BET)-specific surface area of 1,100 m 2 g −1 , and a very narrow pore size distribution centered at 12.5 nm, as determined by the BJH method. This carbon exhibits a specific pore volume of 2.3 cm 3 g −1 . As shown in a representative high resolution SEM image of a fractured surface ( Fig. 1b ), the pores (~12 nm in diameter; in good accord with the BET data) are distributed with no strict long-range order, and are inter-connected. The porous structure can also be observed in the corresponding dark-field STEM image ( Fig. 1c ). Figure 1: Porosity characterization of the 'silica colloidal monolith'-derived mesoporous carbon (SCM). ( a ) Pore size distribution for SCM carbon. Inset: adsorption/desorption isotherm; ( b ) high-resolution SEM image of SCM; ( c ) dark-field STEM image of SCM. ( b , c ) Scale bar=300 nm. Full size image An advantage of SCM as the carbon framework for the sulphur electrode is that the particle size can be controlled by varying the grinding force and duration on the carbon monolith. 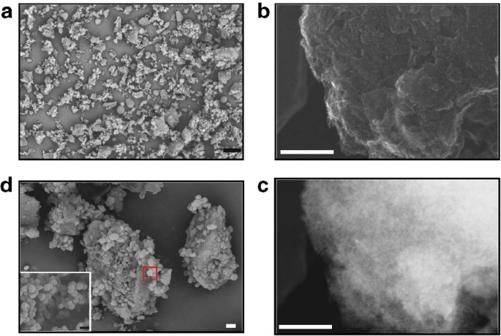Figure 2: Electron micrographs of the SCM/sulphur and SBA-15/SCM/sulphur electrode materials. (a) Low-resolution SEM of SCM, scale bar=20 μm; (b) high-resolution SEM and (c) dark-field STEM images of SCM/S (sulphur 70 wt%). (d) SEM of SCM/S with SBA-15 additive (the white platelets highlighted by the red box), scale bar=1 μm; inset: SBA-15 for reference (scale bar=1 μm). (b,c) Scale bar=300 nm. The SCM used here for the cathode exhibits an irregular morphology and an average particle size of ~10 μm, as shown in the low-resolution SEM image in Figure 2a . The SCM/S electrode will exhibit a higher tap density than counterparts with smaller carbon particle sizes. Importantly, the micron-sized SCM/S structures still preserve all the benefits of nano-dimensions due to their fine porous structure. As shown by the high resolution SEM image in Figure 2b , which can be compared to empty SCM shown in Figure 1c , the surface morphology of SCM is altered after the melt-diffusion process for sulphur impregnation. The corresponding STEM image ( Fig. 2c ) shows much less porosity after sulphur-filling than before ( Fig. 1d ), which is confirmed by pore volume measurements of the SCM/S composite (0.31 cm 3 g −1 ). The particle size of the SCM/S has benefits for electrode preparation as well. Extensive efforts have been devoted to fabricating electrode materials with decreased particle sizes but it has been shown that the superior performance of nanoparticles can come at the expense of necessity of binder overuse, lowered tap density and potential safety concerns [24] . The large particle size of SCM/S means that the amount of the polymer binder necessary to prepare electrodes is reduced to 5 wt% ( vide infra ) compared to the typical content of 20–28 wt% for electrode materials comprising nanoparticles [25] . Thus the composite exhibits the advantage of bulk-sized electrode materials but with internal nanostructure. Figure 2: Electron micrographs of the SCM/sulphur and SBA-15/SCM/sulphur electrode materials. ( a ) Low-resolution SEM of SCM, scale bar=20 μm; ( b ) high-resolution SEM and ( c ) dark-field STEM images of SCM/S (sulphur 70 wt%). ( d ) SEM of SCM/S with SBA-15 additive (the white platelets highlighted by the red box), scale bar=1 μm; inset: SBA-15 for reference (scale bar=1 μm). ( b , c ) Scale bar=300 nm. Full size image Incorporation of the polysulphide 'reservoirs' into the SCM To homogeneously incorporate the silica SBA-15 (10 wt%) within the SCM/S (90 wt%), the solids were well dispersed and mixed by sonication (see Methods ). The platelets are incorporated within the aggregated particles by the mixing process; they are also visible on the surface as shown in the SEM image in Figure 2d . Their characteristic shape makes them easy to identify, which is important for the EDX(Energy dispersive X-ray spectroscopy) studies to verify the sulphur reservoir concept ( vide infra ). 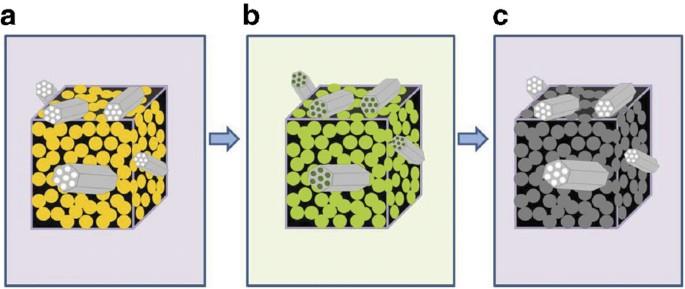Figure 3: Schematic diagram illustrating the concept of the 'polysulphide reservoir' afforded by the SBA-15 platelets in the SCM/S electrode. (a) Before discharge: the black area represents carbon with pores infiltrated by sulphur and grey particles on the cube surface are SBA-15. (b) Discharge to 2.15 V: the green-coloured area denotes polysulphide ions (Sn2−, 3≤n≤8), which are 'concentrated' in the SBA-15. (c) Discharge to 1.5 V: polysulphide ions diffuse out of SBA-15 platelets and are further reduced into solid sulphides (Li2S/Li2S2) within the SCM carbon framework. A schematic that illustrates the incorporation of the SBA-15 into the SCM/S is illustrated in Figure 3a , along with the concept of the function and benefit of the polysulphide reservoirs ( Fig. 3b,c ) that will be discussed in detail later. The electrical conductivity of the electrode materials both with and without the SBA-15 additive was equivalent, ~6 S cm −1 showing that the silica has no effect owing to its low overall concentration. Figure 3: Schematic diagram illustrating the concept of the 'polysulphide reservoir' afforded by the SBA-15 platelets in the SCM/S electrode. ( a ) Before discharge: the black area represents carbon with pores infiltrated by sulphur and grey particles on the cube surface are SBA-15. ( b ) Discharge to 2.15 V: the green-coloured area denotes polysulphide ions (S n 2− , 3≤ n ≤8), which are 'concentrated' in the SBA-15. ( c ) Discharge to 1.5 V: polysulphide ions diffuse out of SBA-15 platelets and are further reduced into solid sulphides (Li 2 S/Li 2 S 2 ) within the SCM carbon framework. Full size image Electrochemistry Electrochemical measurements of SCM/S electrodes were carried out to investigate the influence of the SBA-15 incorporation. 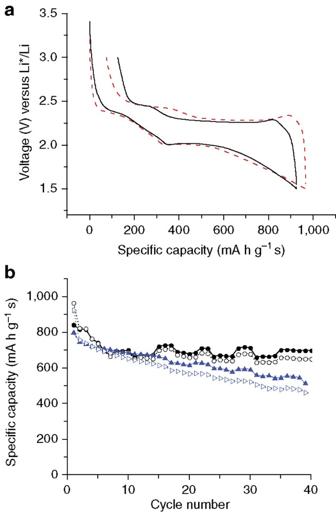Figure 4: Electrochemical data for SCM/S and SBA-15-SCM/S demonstrating the positive effect of silica incorporation. Data were obtained on galvanostatic cycling at a C/5 rate (corresponding to a current density of 334 mA g−1or 0.4 mA cm−2). (a) Comparison of the discharge–charge profiles of the first cycle of SCM/S (black solid line) and SCM/S with the SBA-15 additive (red dotted line). (b) Comparison of the cycling stability of SCM/S (blue) and SCM/S with SBA-15 additive showing the capacity stabilization in the latter case. Discharge capacity: empty symbols; charge capacity: solid symbols. Figure 4a shows the galvanostatic discharge/charge profiles recorded at a current rate of C/5 (334 mA g −1 or 0.4 mA cm −1 ). The initial discharge capacity of the cell with SBA-15 is 960 mA h g −1 , where the mass (g) refers to the active sulphur component, following convention. This is greater than the capacity of 920 mA h g −1 exhibited by the cell without SBA-15. Both cells exhibit some irreversible capacity in the first cycle, but it is less with the SBA-15 additive. It is also evident that cell polarization with SBA-15 is only slightly greater than in the case without it. Overall, the presence of SBA-15 in the sulphur electrode greatly improves the overall electrochemical performance. As Figure 4b (blue curve) shows, without SBA-15, the cell suffers both capacity fading and an increasing divergence between the charge and discharge capacity as a result of the polysulphide shuttle mechanism. It is likely that the large pore size of SCM carbon permits significantly more polysulphide dissolution than CMK-3, for example [15] . With the addition of SBA-15, as Figure 4b (black curve) illustrates, although the cell experiences some initial capacity fading (~30%), from the tenth cycle onward, this is almost completely curtailed. A discharge capacity well above 650 mA·h g −1 is steadily maintained after 40 cycles. Both cells exhibit slightly fluctuating cycling behaviour, which is not yet well understood. We speculate that the release rate of the polysulphide ions from the silica may not be constant, and sudden expulsion may give rise to higher capacity. Further investigation is needed to study this phenomenon. Importantly, the coulombic efficiency is maintained at above 95% for 30 cycles, which indicates the effective suppression of a polysulphide shuttle mechanism in the presence of the SBA-15 additive. Figure 4: Electrochemical data for SCM/S and SBA-15-SCM/S demonstrating the positive effect of silica incorporation. Data were obtained on galvanostatic cycling at a C/5 rate (corresponding to a current density of 334 mA g −1 or 0.4 mA cm −2 ). ( a ) Comparison of the discharge–charge profiles of the first cycle of SCM/S (black solid line) and SCM/S with the SBA-15 additive (red dotted line). ( b ) Comparison of the cycling stability of SCM/S (blue) and SCM/S with SBA-15 additive showing the capacity stabilization in the latter case. Discharge capacity: empty symbols; charge capacity: solid symbols. Full size image Back-of-the-envelope calculations suggest, in fact, that a large fraction of polysulphide can be accommodated in the SBA-15 particles. The theoretical sorption capacity is dependent on whether surface ad sorption or pore ab sorption (or a combination of the two) governs the process. We based our estimate on the assumption of complete dissolution of all of the sulphur in the cathode as polysulphide, which we know does not occur but serves as a boundary point. For the former case—adsorption—a lower limit of about 20% ad sorption is predicted, based on the surface area of the SBA-15 (850 m 2 g −1 ) [26] and that of the intermediate polysulphide S 6 2− species (2.2×10 −19 m 2 /molecule S 6 2− ; see Methods ). In the latter case—absorption—nearly 100% of the polysulphide can be ab sorbed into the volume in the upper limit of complete pore filling (based on the estimated volume of the intermediate polysulphide S 6 2− species of 6.6×10 −29 m 3 /molecule S 6 2− , and a typical pore volume of SBA-15 of 1.2 cc g −1 (ref. 26 ). A reasonable estimate of the sorption capacity lies somewhere between these two extremes. Of course, it is not necessary for SBA-15 to hold all the polysulphide ions at any stage owing to dynamic equilibrium. Therefore, we believe that the fraction of SBA-15 employed in this study is not only valid to demonstrate the concept but adequate to effectively prevent polysulphide ions from diffusing away from the cathode side. To confirm the role of the SBA-15 additive in stabilizing the cycling and its mechanism, we carried out analytical measurements on the electrodes at various stages of cycling. EDX was used to investigate whether electrochemically generated polysulphide anions are absorbed by SBA-15 platelets and desorbed when necessary, that is, near the end of discharge. We employed tetraethylene glycol dimethyl ether as the electrolyte solvent (containing 1 M LiPF 6 ) in the cells for this EDX study and for the analysis of the sulphur concentration in the electrolyte. Elemental analysis could not be performed using the electrolyte based on ethyl methyl sulfone, as it contains sulphur. The concentration of LiPF 6 should be a constant value within SBA-15 particles in the sulphur electrode throughout cycling. The phosphorus signal acts as an internal reference via determination of the S/P ratio. To determine the absorption capacity of SBA-15 additive for polysulphide anions, the electrode material was extracted (in an Ar filled glovebox) from a cell which was discharged to 2.15 V in its 40th cycle at a current rate of C/5 (334 mA g −1 or 0.4 mA cm −2 ). At this potential, elemental sulphur is completely converted to soluble polysulphide species, that is, S 6 2− ·2Li + . The cathode was investigated by SEM and EDX. 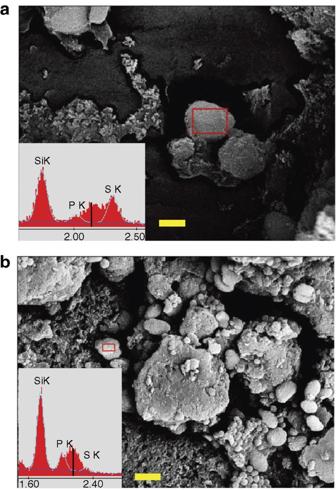Figure 5: SEM and EDX results of the SBA-15-SCM/S electrode at different cell voltages. The EDX results are collected from the area marked by the red boxes shown at the left bottom corner of the images. (a) Discharge to 2.15 V at the 40th cycle reveals an S/P ratio of 3.4, indicating that a high concentration of residual polysulphide is absorbed in the SBA-5 particles. Scale bar=200 nm; (b) Discharge to 1.5 V at the 40th cycle reveals an S/P ratio of 0.2, demonstrating that 94% of the sulphur is released from the SBA-15 at the end of discharge. No glassy sulphide phase is evident on the surface of the particles even after 40 cycles. Scale bar=500 nm. As shown in Figure 5a , EDX signals collected from an SBA-15 particle (marked by the red square) show a very high sulphur/phosphorus (S/P) atomic ratio of 3.4 averaged from 20 spots. Therefore, one can expect that the polysulphide anion concentration in the electrolyte will be much lower in the presence of SBA-15 in the cathode layer, as conceptualized in Figure 3b . This will greatly hinder the redox shuttle in the electrolyte and, in turn, prevent active mass loss on both electrodes. Figure 5: SEM and EDX results of the SBA-15-SCM/S electrode at different cell voltages. The EDX results are collected from the area marked by the red boxes shown at the left bottom corner of the images. ( a ) Discharge to 2.15 V at the 40th cycle reveals an S/P ratio of 3.4, indicating that a high concentration of residual polysulphide is absorbed in the SBA-5 particles. Scale bar=200 nm; ( b ) Discharge to 1.5 V at the 40th cycle reveals an S/P ratio of 0.2, demonstrating that 94% of the sulphur is released from the SBA-15 at the end of discharge. No glassy sulphide phase is evident on the surface of the particles even after 40 cycles. Scale bar=500 nm. Full size image To determine whether the absorbed polysulphide can be desorbed on demand, as schematically illustrated in Figure 3c , electrode material was obtained from another cell which was discharged to 1.5 V at the end of the 40th discharge. A much lower average S/P ratio of 0.2 in the SBA-15 was measured (30 spots), as shown in Figure 5b . By comparing the S/P ratio at 2.15 V and 1.5 V, it is estimated that ~94% of the sulphur mass in the SBA-15 particles was desorbed and participated in electrochemical reactions even during the 40th cycle. Most importantly, we did not observe glassy sulphide agglomeration phase on either electrode surface. Due to the fact that the SBA-15 polysulphide nano-reservoirs reside on the surface of SCM/S particles in addition to being contained within the bulk, polysulphide ions can easily diffuse back within the pores of SCM instead of being reduced on the surface to form agglomerates. The reversible absorption and desorption of polysulphide anions is also facilitated by the insulating properties of the silica. If the absorbent is electronically conductive, we believe that sulphide agglomeration will rapidly occur on the surface of the absorbent. We also measured the sulphur electrolyte concentration in the cells with and without the SBA-15 additive in this large-pore carbonaceous electrode. 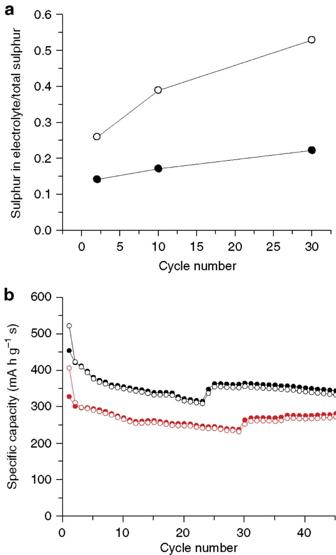Figure 6: Effect of SBA-15 incorporation on sulphur dissolution in electrochemical cells and high-rate cycling behaviour of cathodes. (a) Percentage of sulphur dissolution into the electrolyte from the SCM/S cathode (open symbols); from the SBA-15-SCM/S cathode (solid symbols). (b) Comparison of galvanostatic cycling of SCM/S (black) and CMK-3/S (red) at a current rate of 1C (1,672 mA g−1or 2 mA cm−2), discharge capacity: open symbols; charge capacity: solid symbols. Less than 23% of sulphur is found in electrolyte at 30th cycle in the former case, and 54% of sulphur for the latter case, as shown in Figure 6a . This result confirms the electrochemical results. Figure 6: Effect of SBA-15 incorporation on sulphur dissolution in electrochemical cells and high-rate cycling behaviour of cathodes. ( a ) Percentage of sulphur dissolution into the electrolyte from the SCM/S cathode (open symbols); from the SBA-15-SCM/S cathode (solid symbols). ( b ) Comparison of galvanostatic cycling of SCM/S (black) and CMK-3/S (red) at a current rate of 1C (1,672 mA g −1 or 2 mA cm −2 ), discharge capacity: open symbols; charge capacity: solid symbols. Full size image To confirm the expected good rate performance of SCM/S, we also examined cells at high rates of 1C (1,672 mA g −1 or 2 mA cm −2 ) to compare the SCM/S electrode and a CMK-3/S electrode with the same sulphur loading in the composites (70 wt%), but without the SBA-15 additive. SCM/S shows higher capacity than its CMK-3 counterpart, as shown in Figure 6b . The larger pore size of the carbon structure for C/S electrode is clearly advantageous in high power applications. Interestingly, both cells show no shuttle phenomenon at this C rate and a stable cycling performance. By comparison to Figure 4b (blue curve), it is evident that the coulombic efficiency is improved to about 98% at high current rates. It is likely that dissolution/diffusion is diminished under these conditions. Our results can be compared with other recent studies on Li/S cells where some new approaches have been explored, from two aspects: cycling stability and coulombic efficiency. A good summary of the effect of carbon pore structure is provided by the work of Liang et al ., where a bimodal micro-mesoporous carbon was utilized to increase the carbon absorption capacity of polysulphide ions [14] . Compared with a mesoporous (7 nm) carbon studied in their work, which displayed dramatically rapid capacity fading of 80% over 10 cycles, the bimodal carbon at low sulphur/carbon loading in the composite (11 wt%) exhibited more stable capacity retention of about 50% over 30 cycles. Coulombic efficiency was not provided. Sulphur/carbon ratios in the bimodal carbon up to 52 wt% increased the fade rate to 60% however, which is about double of that we find with the SBA-15 additive. By using a microporous (<0.7 nm) carbon to form a C/S composite, Gao et al . [27] reported very unusual stable cycling performance at a capacity of 800 mAh g −1 with 100% coulombic efficiency. This was based on a very low sulphur loading of 29 wt% of the electrode mass [27] . Higher loading led to extremely low utilization of the active sulphur. The flat, low potential of 1.8 V on the first cycle, the use of carbonate electrolytes and highly sloping subsequent discharge profiles are not characteristic of Li–S cells, however. It suggests that treatment of the S/C composite at 300 °C may have resulted in formation of a C–S polymer or that other factors are at play. In another interesting study, Cui et al . [10] studied the fully discharged form of a S electrode (Li 2 S/CMK-3), with no control on polysulphide diffusion. A clear shuttle phenomenon was observed and the capacity and cycling stability were also poor. Important progress was recently made by Hassoun and Scrosati [9] , who showed that by combining S/C cathodes with lithium sulfide-saturated polymer electrolytes, and Sn/C anodes, a good cycling stability (about a 30% fade rate over 30 cycles), similar to that reported here, could be obtained at low rates (C/20). Comparison is made difficult by the large differences in cell configuration. In summary, we observe that stabilized cycling with a high coulombic efficiency has not been reported for Li–S cells at practical S/C loadings at high rates. Our results fill this void and represent the best level achieved so far to the best of our knowledge. This was made possible by utilizing a mesoporous silica that is shown to be a highly effective internal polysulphide reservoir for the cathode in Li–S batteries. This not only greatly improves the cycling stability but also eliminates the polysulphide shuttle mechanism to a large degree and allows large-pore carbons to be utilized. A mesoporous monolithic carbon with a large particle size around 10 μm and a uniform large mesopore size of 12.5 nm was prepared and investigated as an encapsulating chamber for the sulphur active mass. The C/S composite exhibits larger tap density, less need for binder and very good rate performance. Although we have established proof-of-concept with SBA-15, we expect this approach to be widely applicable to other silicas with suitable mesopores of dimensions large enough to accommodate the polysulphide ions. Key to the polysulphide reservoir concept is that the material permits absorption/desorption in a reversible manner during the electrochemical reaction. Preparation of SCM Silica colloid (LUDOX HS-40 40 wt%, Sigma-Aldrich; 5 g) was dried in a petri dish to form a semi-transparent silica monolith template (2g), which was impregnated for 10 min with an isopropyl alcohol solution (5 ml) containing 80 mg of oxalic acid (97% Fluka), as a catalyst for the polymerization of the carbon precursors. The isopropyl alcohol was then removed by evaporation at 85 °C. The oxalic acid-loaded silica monolith was impregnated in a mixture of 2 g of resorcinol (98%, Sigma-Aldrich) and 1.7 g of crotonaldehyde (98%, Sigma-Aldrich) for 1 h. Filtration was applied to the soaked silica monolith to remove excessive precursor. The mixture was then subjected to polymerization through a series of heat treatments in air under the following conditions: 60 °C for 30 min, 120 °C for 10 h, 200 °C for 5 h. The resultant polymer was carbonized at 900 °C under an argon atmosphere. The silica/carbon composite monolith was ground into a powder before the silica template was removed by HF (15%) etching. Preparation of CMK-3 and the CMK-3/S composite We have followed the same procedures described in our previous paper [15] . CMK-3/S contains 70 wt% of sulphur in the composite. Preparation of SCM/S A mixture of SCM (0.2 g) and sulphur (0.47 g) was ground, and melt diffusion was carried out in an oven at 155 °C. The composite contains 70 wt% of sulphur. Synthesis of SBA-15 Pluronic P123 (EO 20 PPO 70 EO 20 ), 2 g, was dissolved in 60 ml of 2 M HCl solution at 38 °C. Tetraethylorthosilicate (4.2 g) was added to the above solution under vigorous stirring. The mixture was stirred for 6 min and remained quiescent for 24 h at 38 °C. The mixture was subsequently heated at 100 °C for another 24 h in an autoclave. The as-synthesized SBA-15 with platelet morphology was collected by filtration, dried and calcined at 550 °C in air. Preparation of SBA-15–SCM/S composites A mixture of SBA-15 (50 mg) and SCM/S (450 mg) was dispersed in water (5 ml), and sonicated for 30 min and stirred for 2 h. The mixture was then filtered and dried at 80 °C overnight to remove residual water. Electrochemical measurements Positive electrodes were constructed from SCM/S-SBA-15 (95 wt%), and polyvinylidene fluoride (PVDF) binder (5 wt%). The cathode material, ready for electrochemical studies, contained 60 wt% of sulphur as active mass. The cathode material was well dispersed in cyclopentanone by sonication and slurry-cast onto a carbon-coated aluminium current collector (Intelicoat), and 2,025 coin cells were constructed using an electrolyte composed of a 1.2 M LiPF 6 solution in ethyl methyl sulphone. Lithium metal foil was used as the counter electrode. For the electrode containing CMK-3/S, 8 wt% PVDF binder was employed. Only in the comparison study with CMK-3/S was the SCM/S electrode also mixed with 8 wt% of PVDF binder. According to the active mass loading (1.2 mg cm −2 ), the equivalent current density for the 334 mA g −1 rate is 0.4 and that for the 1,672 mA g −1 is 2 mA cm −2 . To measure the degree of sulphur retention in the cathode, a 1.0 M LiPF 6 solution in tetraethylene glycol dimethyl ether was used as the electrolyte. SCM/S-SBA-15 cathodes were compared with SCM/S cathodes containing no SBA-15 at the exact same S/C ratio. We used large Swagelok-type cells that accommodate a sufficient excess of the electrolyte to dissolve sulphur species. Swagelok cells were disassembled and a portion of the electrolyte with the volume accurately measured was taken and diluted for sulphur concentration measurement, which was carried out by Galbraith Laboratories. The total dissolution can be calculated based on measured concentration and the total volume of the added electrolyte, which was recorded when assembling the cell. Characterization Nitrogen adsorption and desorption isotherms were obtained using a Quantachrome Autosorb-1 system at −196 °C. Before measurement of SCM, the sample was degassed at 150 °C on a vacuum line following a standard protocol. It was not possible to carry this out for SCM/S owing to the volatility of the sulphur, and so no pretreatment was used. The BET method was used to calculate the surface area. The total pore volumes were calculated from the amount adsorbed at a relative pressure of 0.99. The pore size distributions were calculated by means of the Barrett–Joyner–Halenda method applied to the desorption branch. The morphology of the SCM/S-SBA-15 composites was examined by a LEO 1530 field-emission SEM instrument equipped with an energy-dispersive X-ray spectroscopy attachment. TEM images in this study were obtained with a Hitachi HD-2000 scanning transmission electron microscope. Calculation of adsorption of polysulphides in SBA-15 The S 6 −2 molecule was used as the prototype polysulphide anion. Gaussian calculations determined the length of the molecule as 7.33 Å and the width as ~3 Å×3 Å. Surface adsorption. The maximum surface area of S 6 −2 in the flat configuration is 2.19×10 −19 m 2 /molecule. Thus, compared with the surface area of SBA-15 (ref. 26 ) of ~850 m 2 g −1 , 6.44×10 −3 mol S 6 −2 can be adsorbed per gram of SBA-15; that is, 1.28×10 −6 mol S 6 −2 , or 7.7×10 −6 mol of sulphur, can be adsorbed in the as-prepared electrodes, which contain ~0.2 mg of SBA-15 (that is, 10 wt%). Compared with the total mass of sulphur in the electrode (1.2 mg), the SBA-15 can therefore accommodate about 20% of the sulphur mass in the extreme lower limiting case of surface adsorption—where the S 6 −2 molecules only adsorb on the surface of SBA-15 utilizing the maximum surface area of their structure, and only monolayer adsorption occurs. 'End' adsorption or bi/trilayer adsorption would double or triple this value. Surface absorption. The volume spanned by the S 6 −2 molecule is approximately 6.57×10 −29 m 3 /molecule, and the typical pore volume of SBA-15 is ~1.2 cm 3 g −1 . Thus, 3.03×10 −2 mol S 6 −2 can be absorbed per gram of SBA-15, or 6.06×10 −6 mol S 6 −2 per electrode given the mass of SBA-15 present (see above). This is equivalent to 3.6×10 −5 mol of sulphur , which, compared with the total mass of sulphur in the electrode, means that the SBA-15 can accommodate about 97% of the sulphur mass in the extreme upper limiting case of pore absorption if complete pore filling occurs. The expected co-adsorption of Li + ions and solvent molecules would decrease this value by perhaps a factor of two or three.